Four-colour FRET reveals directionality in the Hsp90 multicomponent machinery In living organisms, most proteins work in complexes to form multicomponent protein machines. The function of such multicomponent machines is usually addressed by dividing them into a collection of two state systems at equilibrium. Many molecular machines, like Hsp90, work far from equilibrium by utilizing the energy of ATP hydrolysis. In these cases, important information is gained from the observation of the succession of more than two states in a row. We developed a four-colour single-molecule FRET system to observe the succession of states in the heat shock protein 90 (Hsp90) system, consisting of an Hsp90 dimer, the cochaperone p23 and nucleotides. We show that this multicomponent system is a directional ATP-dependent machinery. This reveals a previously undescribed mechanism on how cochaperones can modify Hsp90, namely by strengthening of the coupling between ATP hydrolysis and a kinetic step involved in the Hsp90 system resulting in a stronger directionality. On the single-molecule level the F1-ATPase [1] and the myosin [2] and kinesin [3] families are the best-characterized multicomponent protein machineries. Helicases [4] and gyrases [5] are currently investigated in a similar manner. For all these machines, the sequential succession of many states can be directly observed by measuring the rotation angle or the distance moved, respectively [6] . This cannot be done for the vast majority of biological molecular machines, because they do not step forward or rotate [7] . We demonstrate on the example of heat shock protein 90 (Hsp90) that four-colour single-molecule Fluorescence Resonance Energy Transfer (smFRET) can overcome this limitation by showing the succession of several states independent of stepping. Hsp90 is one of the most abundant proteins in the eukaryotic cell. It supports the folding and maturation of a multitude of client proteins [8] . Many of these clients are involved in cell cycle and regulation, which makes Hsp90 an interesting cancer drug target [9] , [10] , [11] , [12] , [13] . Hsp90 is a dimer consisting of two elongated chains lying in parallel; each chain contains an amino-terminal (N-terminal) ATP binding site [14] , [15] , [16] . Large N-terminal open–close movements of the dimer occur in all investigated Hsp90 systems [17] , [18] , [19] , [20] , [21] , [22] , [23] , [24] , [25] , [26] . Likely, these open–close movements are stronger coupled to ATP hydrolysis in the bacterial Hsp90 (HtpG) compared with the eukaryotic yeast Hsp90, which might raise the question why Hsp90 lost some nucleotide control during evolution from prokaryotes to eukaryotes. A key difference between HtpG and eukaryotic Hsp90 is the existence of small, modifying proteins called cochaperones. Many of them are known to interact with yeast Hsp90, whereas up to now none has been found for HtpG. A current hypothesis is that the control by nucleotides in HtpG has been given up for a much more sophisticated control by cochaperones in eukaryotic Hsp90, making this an example for a multicomponent system. Another puzzle is how two Hsp90 isoforms in the eukaryotic cytosol can enable such a multitude of functions. Previous studies have explained Hsp90’s versatile client recruitment by focusing on how cochaperones affect the conformational equilibrium in Hsp90’s ATPase cycle (for review, see refs 24 , 25 ). 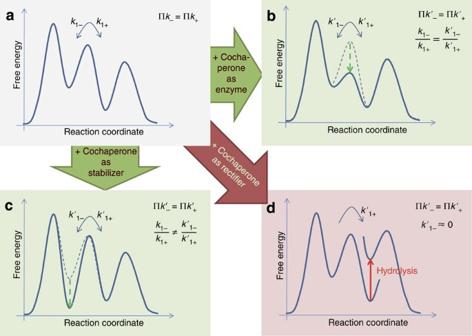Figure 1: Possible mechanisms on how cochaperones act on their chaperone. (a) Free energy of a multistate system in the absence of cochaperones and directionality. (b) Enzyme-like action of a cochaperone: the energy barrier between states is changed, but the equilibrium stays the same. (c) Stabilizing-like action of a cochaperone: the equilibrium between states is changed. (d) Rectifying action of a cochaperone: the number of forward and backward steps is not equal anymore. Figure 1 depicts the possible mechanisms of action of a cochaperone and how they can be distinguished. First, the cochaperone could act as an enzyme and reduce the energy barrier in between some states, not changing the equilibrium. Second, it could act as a ‘stabilizer’, making one or more states relatively more stable and therefore more likely. In both cases, no external energy source is needed. In the third case, the cochaperone induces or changes the directionality of the system. For a directionality, an external energy source like ATP is necessary. The magnitude of the directionality is determined by the coupling strength of hydrolysis to the change in state, which might be modified by the cochaperone. Similar to others [27] , we use the integral over the Gibbs Free Energy G as a quantitative measure for the directionality: Figure 1: Possible mechanisms on how cochaperones act on their chaperone. ( a ) Free energy of a multistate system in the absence of cochaperones and directionality. ( b ) Enzyme-like action of a cochaperone: the energy barrier between states is changed, but the equilibrium stays the same. ( c ) Stabilizing-like action of a cochaperone: the equilibrium between states is changed. ( d ) Rectifying action of a cochaperone: the number of forward and backward steps is not equal anymore. Full size image This is the energy per cycle that is gained or has to be added, respectively. It is zero in the absence of any energy source. T is the temperature, k B the Boltzmann constant and k i+ and k i− are the rates for the i-th forward and backward transition, respectively. Another way to determine directionality is to observe the relative probability for forward and backward transitions for single molecules. If these two probabilities are not the same (that is, there are more transitions from A to B compared with transitions from B to A), there has to be directionality. In the following, we use four-colour smFRET to simultaneously monitor the sequence of states for the conformational changes in Hsp90, the binding of the cochaperone p23 (also called Sba1 in yeast) [28] , [29] , [30] and the binding of ATP. Four-colour single molecule FRET has been utilized before to investigate the movement of DNA holiday junctions [31] , energy transfer paths [32] or Mutα on DNA [33] , but not to address the sequence of events in a multicomponent protein system. Here, we show with four-colour FRET that the cochaperone p23 controls Hsp90 not only by changing the height of energy barriers or shifting the equilibrium of states, but also by increasing the directionality in this non-equilibrium system. We anticipate that this method and analysis will become important for many other multicomponent protein machines. p23 rearranges on Hsp90 during ATP turnover First we determine suitable positions for the fluorophores in the multicomponent system consisting of a yeast Hsp90 dimer, yeast p23 (Sba1) and ATP. The mapping for Hsp90’s conformational changes and nucleotide binding has been done before [22] , and resulted in labelling of ATP at the γ-phosphate and the two Hsp90 monomers at amino acid position 385 in the M-domain and position 61 in the N-domain ( Fig. 2d ). For p23, we tested several positions, mainly position 2 in the N-terminal part ( Fig. 2b ) and position 189 in the unstructured carboxy-terminal (C-terminal) part ( Fig. 2e ). We first probed the energy transfer between an N-terminal labelled Hsp90 and N-terminal (position 2) labelled p23 with Atto488 and Atto594, respectively ( Fig. 2b ). According to X-ray crystallography [14] , isothermal titration calorimetry [34] , NMR and native mass spectrometry [35] we should be able to obtain a high acceptor (orange) signal for binding of p23 to Hsp90 and a low signal for unbinding. Indeed, Fig. 3a shows strong N-terminal contact on the addition of non-hydrolysable AMP-PNP (bottom). Interestingly, we do hardly observe any contact in the presence of ATP (top). In contrast, when the C-terminal part of p23 (which is unresolved in the crystal structure) is monitored together with the M-domain of Hsp90, there is significant binding in the presence of ATP and AMP-PNP, although with different kinetics and a rather low affinity ( Supplementary Figs 1 and 2 ). 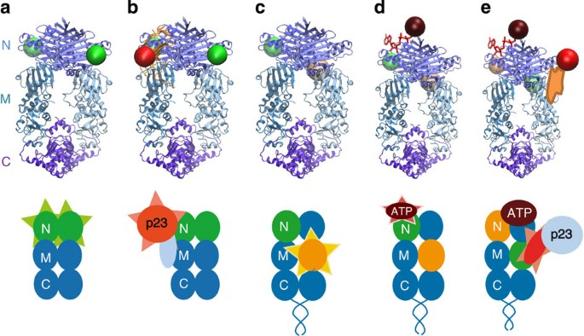Figure 2: Label positions and their visualization. The top row shows the position of the fluorescence labels in the crystal structure (PDB 2CG9) and the bottom row the pictograms used in the following, triangles depict fluorescence. At each configuration, the highest-energy fluorophore is excited. (a) One donor fluorophore (Atto488) in each of the monomers of Hsp90 at position 61. On excitation, both fluorophores will show fluorescence. (b) Same as inawith an additional acceptor (Atto594) in p23 at position 2. The acceptor will show fluorescence on binding. (c) One donor (Atto488) at position 61 in Hsp90 and one acceptor (Atto550) at position 385 in Hsp90. The acceptor will show fluorescence on closing of Hsp90. (d) Same as incwith an additional acceptor (Atto647N) at the γ-phosphate of ATP. The latter will show fluorescence on binding. (e) Same as indwith an additional acceptor (Atto594) at position 189 in p23. The fluorophore on p23 shows fluorescence if all components are together. Figure 2: Label positions and their visualization. The top row shows the position of the fluorescence labels in the crystal structure (PDB 2CG9) and the bottom row the pictograms used in the following, triangles depict fluorescence. At each configuration, the highest-energy fluorophore is excited. ( a ) One donor fluorophore (Atto488) in each of the monomers of Hsp90 at position 61. On excitation, both fluorophores will show fluorescence. ( b ) Same as in a with an additional acceptor (Atto594) in p23 at position 2. The acceptor will show fluorescence on binding. ( c ) One donor (Atto488) at position 61 in Hsp90 and one acceptor (Atto550) at position 385 in Hsp90. The acceptor will show fluorescence on closing of Hsp90. ( d ) Same as in c with an additional acceptor (Atto647N) at the γ-phosphate of ATP. The latter will show fluorescence on binding. ( e ) Same as in d with an additional acceptor (Atto594) at position 189 in p23. The fluorophore on p23 shows fluorescence if all components are together. 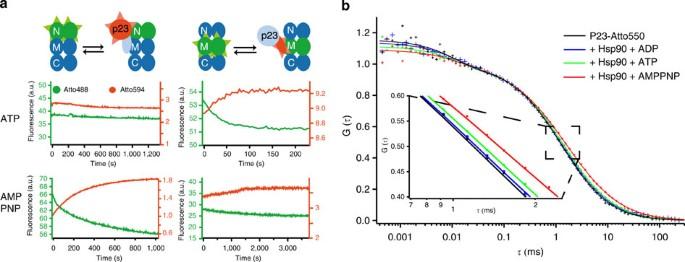Figure 3: p23 rearranges during ATP turnover of Hsp90. (a) Ensemble FRET measurements of p23 binding to Hsp90. Binding between the N-terminal domains of Hsp90 and p23(left) in the presence of AMP-PNP (bottom) or ATP (top) is compared with binding between the C-terminal part of p23 and the M-domain of Hsp90 (right). (b) FCS curves of 1 nM-labelled p23 in the absence of Hsp90 and in the presence of 10 μM Hsp90 and 2 mM ADP, 2 mM ATP or 2 mM AMP-PNP, respectively. Each curve is scaled, such that the mean number of molecules in the volume isN=1 in each case. The fits result in a mean diffusion time oftp23-only=1.31±0.02 ms,tADP=1.33±0.02 ms,tATP=1.44±0.02 ms andtPNP=1.81±0.05 ms, respectively. Errors are the s.d. of four independent measurements each. See Methods for details. Both complementary methods result in very similar nucleotide dependent affinities and thus confirm the proposed mechanism of the Hsp90–p23 machinery. Full size image Figure 3: p23 rearranges during ATP turnover of Hsp90. ( a ) Ensemble FRET measurements of p23 binding to Hsp90. Binding between the N-terminal domains of Hsp90 and p23(left) in the presence of AMP-PNP (bottom) or ATP (top) is compared with binding between the C-terminal part of p23 and the M-domain of Hsp90 (right). ( b ) FCS curves of 1 nM-labelled p23 in the absence of Hsp90 and in the presence of 10 μM Hsp90 and 2 mM ADP, 2 mM ATP or 2 mM AMP-PNP, respectively. Each curve is scaled, such that the mean number of molecules in the volume is N =1 in each case. The fits result in a mean diffusion time of t p23-only =1.31±0.02 ms, t ADP =1.33±0.02 ms, t ATP =1.44±0.02 ms and t PNP =1.81±0.05 ms, respectively. Errors are the s.d. of four independent measurements each. See Methods for details. Both complementary methods result in very similar nucleotide dependent affinities and thus confirm the proposed mechanism of the Hsp90–p23 machinery. Full size image These observations can be explained by p23 binding to the middle domain of Hsp90 in the presence of ATP and rearrangement to the N-domain of Hsp90 directly before ATP hydrolysis (AMP-PNP state). In addition, a fast release of p23 after hydrolysis would be required, because there is no significant change in fluorescence of the N-terminal labelled species on the addition of ATP. We confirmed this by fluorescence correlation spectroscopy (FCS). P23 is labelled at position 66 with Atto550 and its diffusion time determined in absence and presence of unlabelled Hsp90 and various nucleotides. Figure 3b shows indeed that in the presence of ADP and Hsp90 we observe nearly the same diffusion time as in the absence of Hsp90, that is, practically no binding to Hsp90. Clear binding is observed in the presence of ATP and even more in the presence of AMP-PNP, indicated by an increasing mean diffusion time. Therefore, p23 is released from the ATP to the ADP state. Finally, we excluded that the fluorophore causes the affinity of labelled p23 to labelled Hsp90 ( Supplementary Fig. 3 ). Altogether this might explain why ATP-γS strongly populates the N-domain closed state of Hsp90 in the presence of p23, but ATP does not [18] , namely by a previously unreported rearrangement of p23 on Hsp90 between the initially ATP bound state and the ATP hydrolysis state (which is usually probed by AMP-PNP or ATP-γS). p23 accelerates the binding of ATP to Hsp90 In the following, we quantify how the presence of p23 impacts ATP binding to Hsp90. To that aim, twofold labelled Hsp90 (Atto488, Atto550) was measured in the presence of labelled ATP (Atto647N) and in the presence or absence of labelled p23, for schematic and more details, see Fig. 4a . This four-colour assay is further refined in the next section to use the full four-colour information. Here, we focus on the two dyes at Hsp90 and the label at the ATP. 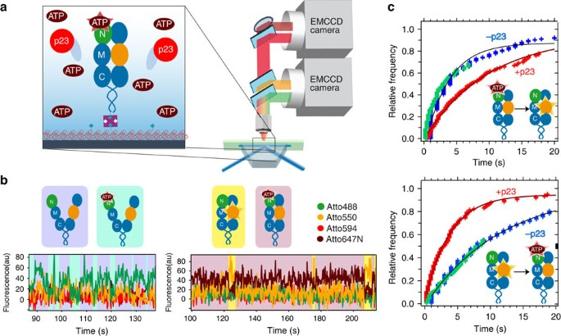Figure 4: p23 accelerates the binding of ATP to Hsp90. (a) Schematics of the single-molecule four-colour FRET experiment with a single Hsp90 dimer labelled with Atto488 and Atto550, 500 nM p23 N-terminally labelled with Atto594 and 200 nM ATP labelled with Atto647N. (b) Example traces for the binding of ATP to the open (left) and closed (right) state of Hsp90, p23 binding is discussed in the next figure. (c) Cumulative histograms of dwell times with ATP bound (top) and unbound (bottom). Red crosses are in the presence of p23, while green and blue crosses are in the absence of p23 (220 ms and 1,000 ms time resolution, respectively). Data are normalized to one, lines show exponential fits, a total of 200 traces were observed (seeSupplementary Notes, page 16 for details). Figure 4b shows two example traces for ATP binding to the open and close states of Hsp90, respectively (see Supplementary Fig. 4 for a more detailed view of these traces). With the help of Hidden Markov Analysis (HMM, see Supplementary Fig. 5 for HMM traces) we obtained the dwell time distributions for the binding of ATP to the closed state of Hsp90 as shown in Fig. 4c . The binding to the closed state is clearly stabilized by the presence of p23, whereas ATP binding in the open state remains unaffected ( Supplementary Fig. 6 ). See Supplementary Fig. 7 for 2D-histograms for ATP binding/unbinding in the presence and absence of p23. Interestingly, p23 is at the same time stabilizing the ATP bound state and accelerating the binding of ATP. ATP unbinding from the closed state in the absence of p23 seems to be biphasic and a double exponential fit (four fit parameters) matches the data better. Interestingly, the obtained longer dwell time fits well with the dwell time in the presence of p23. We cannot discuss this further at this point, because a power law with only three fit parameters would also fit the data well. Figure 4: p23 accelerates the binding of ATP to Hsp90. ( a ) Schematics of the single-molecule four-colour FRET experiment with a single Hsp90 dimer labelled with Atto488 and Atto550, 500 nM p23 N-terminally labelled with Atto594 and 200 nM ATP labelled with Atto647N. ( b ) Example traces for the binding of ATP to the open (left) and closed (right) state of Hsp90, p23 binding is discussed in the next figure. ( c ) Cumulative histograms of dwell times with ATP bound (top) and unbound (bottom). Red crosses are in the presence of p23, while green and blue crosses are in the absence of p23 (220 ms and 1,000 ms time resolution, respectively). Data are normalized to one, lines show exponential fits, a total of 200 traces were observed (see Supplementary Notes , page 16 for details). Full size image p23/Hsp90 is directional and coupled to ATP hydrolysis The presented results rule out a purely enzymatic action of p23 as the equilibrium is shifted. They could still be explained with a stabilizing action of p23, if there was no directionality. To decide if there is any directionality in the p23/Hsp90 system, we developed the four-colour FRET system depicted in Fig. 5a . Double-labelled Hsp90 heterodimers were encapsulated in vesicles together with C-terminally labelled p23 in the presence of labelled ATP. From the obtained four-colour fluorescence curves (example curves in Fig. 5b and Supplementary Figs 8 and 9 ), the time-resolved relative distances between the fluorophores and therefore the kinetic steps involved can be extracted. For details on data processing, see Supplementary Notes, page 14ff . In the following, we discuss the fluorescence curves that show p23 and ATP binding events. We obtain a binding time for p23 of 12 seconds as a lower limit, because p23 binds often longer than the time until photo-degradation of the fluorophore ( Supplementary Fig. 10 ). Moreover from these FRET curves the sequence of binding processes can be obtained (see Supplementary Notes, page 17 , for details). We have determined the succession of states for 48 traces showing at least one p23 binding event (see table 1 ) and obtain clearly unequal values for the forward and backward probabilities (the 95% confidence interval by Clopper and Pearson [36] is given in Table 1 ). The prevalent directed succession of states can be seen in Fig. 5c : closed apo state (1)→ ATP binding (2)→ p23 binding (3)→ (ATP hydrolysis and loss of Phosphate) -> loss of p23 → closed apo state (1). 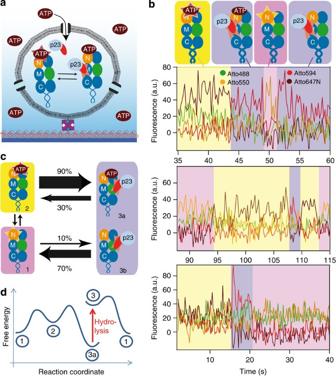Figure 5: The Hsp90/p23 system is directed and coupled to ATP hydrolysis. (a) Schematics of the four-colour FRET measurement with a twofold labelled Hsp90 heterodimer (Atto488, Atto550) and labelled p23 (Atto594) encapsulated in vesicles with a radius of around 100 nm, which contain α-hemolysine pores that allow entering of labelled ATP (Atto647N, 200 nM). (b) Example curves showing different types of transitions as depicted by the colour code. (c) Approximate values for the relative frequency (probability) of the observed transitions. Exact values and confidence intervals are given inTable 1. (d)Relative energy of the different states estimated from the transition probabilities (Table 1) and the occupancy of the states (Supplementary Fig. 7), formula seeSupplementary Notes, page 18. The state after hydrolysis is called state 3 (the sum of all p23 bound states), as we cannot tell at what stage the energy of hydrolysis is utilized (hydrolysis, Pi or ADP release). Estimates: ΔG1->2=1.1kBT; ΔG2–>3a=−2.4kBT; ΔG3a–>3=4.9kBT; ΔG3–>1=−3.6kBT. As a measure for the directionality we obtain from equation (1) for the rate constant from state i to j being k i->j (for details see the Supplementary Notes , page 17): Figure 5: The Hsp90/p23 system is directed and coupled to ATP hydrolysis. ( a ) Schematics of the four-colour FRET measurement with a twofold labelled Hsp90 heterodimer (Atto488, Atto550) and labelled p23 (Atto594) encapsulated in vesicles with a radius of around 100 nm, which contain α-hemolysine pores that allow entering of labelled ATP (Atto647N, 200 nM). ( b ) Example curves showing different types of transitions as depicted by the colour code. ( c ) Approximate values for the relative frequency (probability) of the observed transitions. Exact values and confidence intervals are given in Table 1. (d) Relative energy of the different states estimated from the transition probabilities ( Table 1 ) and the occupancy of the states ( Supplementary Fig. 7 ), formula see Supplementary Notes , page 18. The state after hydrolysis is called state 3 (the sum of all p23 bound states), as we cannot tell at what stage the energy of hydrolysis is utilized (hydrolysis, Pi or ADP release). Estimates: ΔG 1->2 =1.1 k B T ; ΔG 2–>3a =−2.4 k B T ; ΔG 3a–>3 =4.9 k B T ; ΔG 3–>1 =−3.6 k B T . Full size image Table 1 Transition probabilities and 95% confidence intervals according to Clopper and Pearson. Full size table Or for the probabilities p: Such a directionality requires an external energy source [27] , [37] . Thus, the observed reaction cycle has to be coupled to ATP hydrolysis. Finally, the obtained probabilities and rate constants allow us to estimate the relative energy difference between the different states ( Fig. 5d ). A cochaperone could impact the main chaperone either in an enzyme-like fashion or by stabilizing a certain state or by modifying its directionality ( Fig. 1 ). Our newly designed four-colour smFRET system allows to directly distinguishing these three cases. We find that Hsp90 and p23 form a multicomponent machine, with nucleotide turnover causing rearrangements of the binding partners ( Fig. 3 ) in a directional manner ( Fig. 5 ). The main function of ATP turnover is likely to switch the affinities of the different p23 binding sites and not a direct impact on the large N-terminal conformational changes in the Hsp90 dimer. Our findings are largely consistent with previous literature. First, several cycles for Hsp90 with cochaperones (including p23) have been suggested before, for review, see ref. 24 . These cycles suggest directionality in the multicomponent system from the indirect evidence that ATP is hydrolysed. Here, we have directly shown and quantified directionality in the Hsp90/p23 system. In the following, we compare quantitatively the measured directionality to another cycle in the Hsp90 system in the absence of p23. The cycle for the N-terminal open–close movement has recently been solved [22] . Putting the numbers from this publication into equation (1) we obtain a ‘directionality’ of around 1 k B T . This is the thermal energy and therefore consistent with the finding, that idle Hsp90 is mainly dominated by thermal fluctuations. Here we find that in the presence of p23 the directionality is more than 3 k B T . This is significantly higher compared with the thermal energy, although less than one-sixth of the energy from ATP hydrolysis (around 20 k B T ). The absolute values for the directionality in a cellular system might be different for two reasons. First they might be biased by the labels and second by the higher cellular p23 concentrations. In our measurements, we have to operate at low p23 concentration, where only one p23 binds at a time, while likely two p23 are bound at higher concentrations—at least in the presence of AMP-PNP. Please note that stronger coupling does not imply an acceleration of ATP hydrolysis. In fact, a reduction in ATP hydrolysis rate as determined by several labs [34] , [38] is consistent with our model, because the ATPase rate is likely limited by a conformational change prior to ATP hydrolysis, and not by ATP hydrolysis itself (for review, see ref. 24 ). Our results clearly show that p23 is asymmetric; the binding of the first p23 has a different affinity compared with the second p23. Therefore, our results support previous findings showing that asymmetry plays an important role in homodimeric Hsp90 systems: asymmetry is required for client binding [39] , asymmetric SUMOylation facilitates cochaperone binding [40] , nucleotide affinity is asymmetric [22] and hydrolysis is only required in one subunit [41] , [42] . In addition, our data supports the speculation that the loss of directionality from bacterial to yeast Hsp90 is (partly) regained by cochaperones (here: p23). This does not contradict previous studies, which show that nucleotide binding (ADP or AMP-PNP, and therefore not necessarily hydrolysis) shifts the open–close equilibrium across species [26] , as a shift in equilibrium (population) need not be coupled to ATP hydrolysis (see Fig. 1 ). A reason for loss in nucleotide control might be that a control by nucleotides is limited to few conformational states (apo, ATP, ADP.P, ADP or P), while a multicomponent machine that is controlled by both nucleotides as well as the large variety of cochaperones likely results in a much more sophisticated control, which might be advantageous in the more complex eukaryotic cell. This might in turn explain how two Hsp90 isoforms in the eukaryotic cytosol can enable such a multitude of functions, in contrast to motor proteins, where dozens of isoforms are available for the different functions. Our new findings on the function of cochaperones are complementary to previous explanations, which focused on how cochaperones affect the conformational equilibrium in Hsp90’s ATPase cycle [24] . Our study hints towards a more complicated mutual interaction between Hsp90 and its cochaperones, which is supported by molecular dynamics simulations [43] . On the basis of experiments, such a mutual interaction has already been suggested for E. coli Hsp90 (HtpG) and a model substrate protein [44] . We anticipate that an extension of our study to other cochaperones will shed new light on the function of Hsp90’s ATPase rate, which is still largely unknown, but which is manipulated in several Hsp90 drugs in clinical studies. Apart from the Hsp90 system, in the living cell, many machines consist of several binding partners forming intermediate complexes in a nucleotide controlled way. Especially in signal transduction and cell regulation they play a crucial role. Examples are G protein-coupled receptors and cyclin-dependent kinases. Thus, the here described multicomponent machine mechanism might be a stereotype for this type of interactions and the presented four-colour smFRET assay deliver the technique to investigate those systems. In addition, this kind of experiments is suited to determine affinities in a multicomponent system with high precision and therefore complements standard pull down and mass spectroscopy experiments. Molecular biology and protein expression/purification Hsp90 constructs As in our previous studies, we used the yeast Hsp90 C-terminal Zipper constructs yHsp90 61C and yHsp90 385C for the single molecule experiments and the same constructs without zipper for the ensemble experiments ( Figs 2a, b , 3a ). Heterologous expression was done in E. coli and purification was done via Ni NTA, ion exchange and size exclusion chromatography [22] . p23/Sba1 cloning and mutations Sba1 encodes a yeast Hsp90 cochaperone that is homologous to vertebrate p23 (ref. 45) [45] . Therefore, both p23 and Sba1 are commonly used to refer to the same yeast Hsp90 cochaperone. In the following, we use p23 as denotation. For easier purification, a His-Sumo-p23 construct was used. The His-SUMO sequence can be cut off by the corresponding protease Senp. Thus, only the native Tag-free protein remains [46] . The corresponding DNA, sequence optimized for expression in E. coli , was synthesized by Life Technologies (Darmstadt, Germany). This sequence was cloned into a pET28 vector (Novagen, Merck, Darmstadt, Germany). The cysteine and amber stop codon point mutations were done with Quick Change Lightning (Agilent Technologies, Santa Clara, USA) according to the supplier’s protocol. The following mutants were used p23 2C, p23 66pAcF (see below), p23 189C. For the cysteine mutants, the natural cysteine in p23 was replaced by serine. Expression and purification of cysteine mutants of p23 Expression and purification were done with the same protocol used for Hsp90 (ref. 23) [23] . With the exception that after the first HisTag purification the His-SUMO-p23 construct was dialysed against 50 mM sodiumphosphate, 200 mM NaCl, 20 mM imidazole, pH 7.8 buffer in presence of 1/100 mol Senp overnight at 4 °C to cut off the HisTag-SUMO sequence. Afterwards, the cleaved protein was applied to a second HisTag column, which allows only cleaved HisTag free protein to flow through. Expression and purification of p23 p-Acetylphenylalanine The system used for unnatural amino acid incorporation has been developed in the Peter Schultz lab [47] . We are particularly thankful to Edward Lemke (EMBL) for helpful advice. The para-Acetylphenylalanine (pAcF) was obtained from Synchem, Felsberg, Germany. Also in this case, a N-terminal HisTag followed by a SUMO cleavage site was used and the corresponding gene synthesized by Life Technologies. This construct was cloned into a pET28 vector and a TAG amber stop codon was introduced by site-specific mutagenesis as described above. The resulting vector was co-transformed with the pAcF pEvol vector which was obtained from the Lab of Peter Schultz, Scripps [48] into BL21 Star cells (Life Technologies). The cells were grown to an OD of 3 at 37 °C in terrific broth medium at high shaking velocities (250 r.p.m. at 2 inch orbit or 310 r.p.m. at 1 inch orbit). They were cooled down to 30 °C and after 1 h, 10 mM pAcF and 0.02% L-Arabinose was added. After another hour, 1 mM isopropyl-β-D-1-thiogalactopyranoside was added. The incubation was run at least 18 h. The purification was done as for the p23 cysteine mutants described above. Labelling All dyes were obtained from AttoTec, Siegen, Germany. All other chemicals were obtained from Sigma Aldrich, Taufkirchen, Germany. Labelling of the cysteine mutants Fluorescent dyes with a maleimide moiety were used for labelling of the proteins. The maleimide allows specific attachment to cysteines that were introduced by site-directed mutagenesis (see above). Labelling was done in the presence of 5–10 mM TCEP and maximal threefold dye excess. The unreacted dye was removed by dialysis against measurement buffer (see below) for at least 2 days at 6 °C (ZelluTrans/Roth Mini-Dialyzer MWCO 12000, Roth). Labelling of the pAcF mutants The labelling was performed with hydroxylamine derivate Atto594. The p23 was transferred into 50 mM potassium acetate, 150 mM KCl, pH 6.0 with a concentration of at least 200 μM. Afterwards, TCEP was added to a final concentration of 2 mM. The sample was degased in vacuum for 10 min and 1 mM dye and 10 mM aniline were added. The reaction sample was brought into nitrogen atmosphere and incubated 2 days at 6 °C. The sample was dialysed against measurement buffer for three days. A rather low degree of labelling of around 20% was obtained. Further lowering the pH or increasing the temperature lead to precipitation of the protein, even though p23 is a very stable protein. Surface fixation For direct surface fixation, N-hydroxysuccinimide-derivated biotin was bound to the proteins, allowing a binding to the surface of the measurement chamber in presence of streptavidin [19] , the non-reacted biotin was removed by dialysis as described for the dye above. Surface fixation in vesicles was done as described in ref. 22 and below. FRET setup All single-molecule measurements were done with a four-colour FRET setup containing four excitation lasers at 473 nm (Cobolt Blues, Cobolt, Solna, Sweden), 532 nm (Compass 215 M, Coherent, Santa Clara, USA), 594 nm (Cobolt Mambo, Cobolt, Solna, Sweden) and 635 nm (Lasiris, Stocker Yale, Quebec, Canada). The lasers are all passed through clean up filters (all filters in this setup are from AHF Analysetechnik, Tübingen, Germany) expanded twofold and led through mechanical shutters. Afterwards, the lasers are overlaid and passed through an acusto-optical tunable filter AOTF, AOTFnC-Vis-Tn, AA Opto-Electronic, Orsay, France). The beam is directed to the measurement chamber and totally reflected. On the opposite site of the measurement chamber, an Apo TIRF × 60, 1.49 NA, oil objective (Nikon, Tokyo, Japan) is used for collecting the fluorescence light. First the collected light goes through a Kepler telescope. In the middle of the telescope, a rectangular area is cut out of the detection beam with half the size of the camera chip. After that, the light is separated via dichroic mirrors and filtered. In every channel, there is a separate lens to focus the fluorescence light onto the camera. Those lenses are placed on translational stages, which allow the focusing of every channel independently. This construction is crucial to overcome the problem that different colours have different focal distances and thus cannot be focused on the camera chip with one shared lens. Two cameras (Andor iXon, Andor, Belfast, Ireland) were used with two colour channels on each camera, with a lateral offset between the two channels. Thus, the same area of the measurement chamber is displayed four times, but for four different colours. To block scattered laser light of the green laser, which would go directly into the green detection channel, a shutter is installed in that detection pathway. This shutter is closed when the green laser is switched on. A scheme of the whole setup is shown in Supplementary Fig. 11 . For measurements with this setup two cameras, mechanical shutters for each laser, the shutter in the detection pathway and the AOTF have to be controlled precisely. Since this was not possible with the AndorIQ software (Andor, Belfast, Ireland), a PCIexpress card with an external clock (PCIe-6535, National Instruments) was used that could be controlled by a self-written software based on LabView (LabView11, National Instruments, Austin, USA). This programme in combination with the PCIe card allows generating all types of trigger patterns at multiple channels. Usually, prism-type TIRF setups are used in combination with water immersion objectives since the sample is fixed to the measurement chamber surface opposite to the objective, which leads to the problem of large object distances. To combine some advantages of prism-type TIRF and oil immersion objectives, we use very thin measurement chambers with a thickness of around 20 μm. To achieve this, polyurethane film (Tegaderm, 3 M, St Paul, USA ) has been used as spacer between a polyethylene glycol-passivated microscopy slide and a coverslip. The tegaderm is self-adhesive on one side. On the other side, spray adhesive (HighTac, Ghiant, Beerse, Belgium) was applied and dried out completely. The spacers are cut out of the adhesive coated Tegaderm and placed between the slide and coverslip. The whole sandwich is heated up to 70 °C, pressed together and cooled down under pressure. Measurements All measurements were done in measurement buffer: 40 mM Hepes, 150 mM KCl, 10 mM MgCl 2 , pH 7.4. Ensemble measurements All bulk measurements were done at RT on a Jasco FP 6500 or FP8500 spectrafluorometer (Jasco Labor- und Datentechnik, Gross-Umstad, Germany), respectively. The different fluorimeters had different scaling of the fluorescence signal resulting in different scaling in Fig. 3 . For rescaled data, see Supplementary Fig. 12 . FRET ensemble measurements Hsp90–p23 interaction For measuring the interaction of the N-terminal part of p23 with the N-terminal part of Hsp90, p23 2C labelled with Atto594 and Hsp90 61C labelled with Atto488 were used. The Atto488 was excited at 490 nm and detected at 530 nm; the Atto594 was detected at 630 nm. For the measurement with AMP-PNP, 1 μM of Hsp90 was mixed with 0.5 μM p23 and 2 mM AMP-PNP were added. For the measurement with ATP, 0.5 μM Hsp90 were mixed with 3 μM p23 and 2 mM ATP were added. For FRET measurements of the interaction of p23's C-terminal part and the middle domain of Hsp90, p23 189C and Hsp90 385C were used. Hsp90 (0.5 μM) were mixed with 2 mM AMP-PNP or 2 mM ATP, respectively, and 3 μM p23 were added. Fluorescence anisotropy measurements p23 2C and 189C labelled with Atto594 were used with 1 μM concentration in all cases. Excitation was at 590 nm and detection at 630 nm. ATP (2 mM) or 2 mM AMP-PNP were added and incubated at room temperature until a stable anisotropy signal was obtained. Afterwards, Hsp90 with a C-terminal Zipper was added stepwise. Four-colour measurement of ATP binding in the presence of p23 The measurement was done as described in ref. 22 with additional 2.5 mM sodium ascorbate and 500 nM p23 66pLys. Only 100 nM p23s were labelled since the click labelling resulted only in around 20% labelling efficiency (see above). Four-colour measurement of ATP and p23 binding in vesicles Hsp90 61C and Hsp90 385C both with a C-terminal Zipper were labelled with Atto550 and Atto488, respectively. The labelled homodimers were exchanged to form heterodimers by mixing them at 47 °C at a monomer concentration of 1.2 μM each label type [19] . Exchange was done in the presence of 0.5 mg ml −1 bovine serum albumin. After the exchange, 1.6 μM p23 189C labelled with Atto594 and 2 mM AMP-PNP and another 0.5 mg ml −1 bovine serum albumin were added. This mixture was incubated 30 min at RT. The vesicle encapsulation was done as described in ref. 22 : 30 μl lipid emulsion in measurement buffer (4 mg ml −1 1,2-dipentadecanoyl-sn-glycero-3-phosphocholine with 1% (mol:mol)1,2-dipalmitoyl-sn-glycero-3-phosphoethanolamine-N-(cap biotinyl) (both from Avanti Polar Lipids, Alabaster,USA)) were added and the solution was extruded with a mini extruder (Avanti Polar Lipids)) and a 100-nm pore membrane. The vesicles were fixed onto a measurement chamber. Afterwards, 5 μM α-hemolysine (Sigma Aldrich, Taufkirchen, Germany) was added and incubated for 1 h at 30 °C. The α-hemolysine was flushed out and 200 nM ATP 647N labelled at gamma position was flushed in. The measurement was done at 30 °C. FCS measurements FCS was done as follows: Free diffusing p23-molecules labelled with Atto550 were measured in a homebuilt confocal microscope similar to other published setups [49] , [50] , [51] . Time traces of photons were recorded with a single photon avalanche photodiode (PDM-50 μm, PicoQuant) for green fluorescence detection and a commercial data acquisition system (HydraHarp 400, PicoQuant) with a picosecond time resolution. The diffusion time τ d can be extracted from the fit of the correlated data using the following equation [52] , [53] : The triplet time described by the first part of the equation is only used to obtain an optimized fit but will not be considered for analysis in this paper. Keeping the geometrical parameter κ constant for each fit, the relative diffusion time τ d through the confocal volume can be extracted from the fit parameters. According to Stokes’ law, the diffusion time is directly proportional to the hydrodynamic radius of the protein-complex. The fraction of bound and unbound p23 to Hsp90 depends on the affinity of p23 to the different states of Hsp90. Using an equation with two diffusion times and two fractions for the fit would be the method of choice if the diffusion time differed by one order of magnitude. The diffusion time of the p23–Hsp90 complex is approximately two times higher than unbound p23. Therefore in this case the mean diffusion time is determined. How to cite this article: Ratzke, C. et al. Four-colour FRET reveals directionality in the Hsp90 multicomponent machinery. Nat. Commun. 5:4192 doi: 10.1038/ncomms5192 (2014).